A dual role for autophagy in a murine model of lung cancer Autophagy is a mechanism by which starving cells can control their energy requirements and metabolic states, thus facilitating the survival of cells in stressful environments, in particular in the pathogenesis of cancer. Here we report that tissue-specific inactivation of Atg5 , essential for the formation of autophagosomes, markedly impairs the progression of KRas G12D -driven lung cancer, resulting in a significant survival advantage of tumour-bearing mice. Autophagy-defective lung cancers exhibit impaired mitochondrial energy homoeostasis, oxidative stress and a constitutively active DNA damage response. Genetic deletion of the tumour suppressor p53 reinstates cancer progression of autophagy-deficient tumours. Although there is improved survival, the onset of Atg5- mutant KRas G12D -driven lung tumours is markedly accelerated. Mechanistically, increased oncogenesis maps to regulatory T cells. These results demonstrate that, in KRas G12D -driven lung cancer, Atg5-regulated autophagy accelerates tumour progression; however, autophagy also represses early oncogenesis, suggesting a link between deregulated autophagy and regulatory T cell controlled anticancer immunity. Macroautophagy (here referred to as ‘autophagy’) involves the sequestration of portions of the cytoplasm in double-membraned vesicles, the autophagosomes, which then fuse with lysosomes to generate autolysosomes, in which the autophagic cargo is degraded by catabolic hydrolases [1] , [2] , [3] . Autophagy allows cells to degrade their own proteins and organelles to maintain cellular homoeostasis required for normal growth and development, the short-term adaptation to stress as well as for the long-term survival of optimally fit cells [1] , [2] , [3] . Deregulations of autophagy have been implicated in multiple degenerative diseases, aging and cancer [4] , [5] , [6] , [7] . In the context of cancer, autophagy can be disabled by oncogenic processes (such as activation of the PI3K-PKB/Akt-mammalian target of rapamycin pathway, overexpression of anti-apoptotic multidomain proteins from the Bcl-2 family or accumulation of mutant p53 protein in the cytosol), and suppression of autophagy constitutes a potentially oncogenic event [8] , [9] . Thus, the inhibition of autophagy provokes genomic instability (for instance, by the failure to destroy micronuclei containing lagging chromosomes) [10] , [11] , interferes with cellular differentiation (owing to the persistence of the midbody remnant, which is usually cleared by autophagy) [12] , affects the propensity of cells to activate senescence programmes [13] , [14] and perturbs cellular metabolism (in part due to the accumulation of malfunctioning mitochondria) favouring the Warburg phenomenon [15] . Although autophagy is frequently disabled at early steps of oncogenesis, it tends to be reinstated at later states of tumour progression, thus allowing the tumour cells to cope with endogenous stress (such as hypoxia) and increasing resistance against chemotherapy or radiotherapy [16] . The relationship between the Ras oncogenes and autophagy are particularly complex. When introduced into normal, untransformed cells, sustained activation of oncogenic HRas or KRas stimulate autophagy, which is then required for long-term cell survival and oncogenic transformation, presumably through the avoidance of cellular senescence [17] or the maintenance of a functional pool of mitochondria and additional bioenergetic effects [18] , [19] . However, acute transgene-enforced overexpression of oncogenic RAS can induce a cytotoxic level of autophagy, and depletion of several genes essential for autophagy, namely, Atg5, Atg7 or Beclin 1, avoid the demise of Ras-expressing cells [20] , [21] . Conversely, in established tumours, the Ras/PI3K/mammalian target of rapamycin signalling pathway may suppress autophagy, and inhibition of Ras then elicits cytoprotective autophagy [22] . The molecular circuitries through which de novo activation of Ras elicits autophagic stress that may either favour or avoid cell death, contrasting with the inhibition of autophagy by the sustained presence of oncogenic Ras in malignant cells, are elusive. Moreover, the impact of autophagy on Ras-induced oncogenesis in vivo is still poorly characterized. We decided to explore the role of autophagy in KRas G12D —elicited lung carcinogenesis, taking advantage of a genetic model in which an adenovirus expressing the Cre recombinase can activate the KRas G12D oncogene in pneumocytes [23] and optionally delete the essential autophagy gene Atg5 (ref. 4 ). We deliberately chose to regulate autophagy by modulating Atg5 expression because this gene is essential for the initiation of autophagy [4] , [24] and its expression levels correlate with autophagy in human tumours [25] , [26] . Here we report the systematic comparison of autophagy-competent ( Atg5 -expressing) and autophagy-deficient ( Atg5 -deleted) KRas G12D lung cancers. While autophagy deficiency accelerates initial oncogenesis, it reduces progression from adenomas to adenocarcinomas, revealing a dual role of autophagy in the oncogenic process. The acceleration of early oncogenesis caused by Atg5 deficiency could be explained by altered immunosurveillance against autophagy-deficient cancer cells. Prolonged lung cancer survival of autophagy-deficient mice To examine the role of autophagy in lung cancer, we introduce an Atg5 floxed/floxed mutation into Lox-Stop-Lox-KRas G12D mice (termed KRas;Atg5 fl/fl hereafter); Atg5 is essential for the formation of autophagosomes [1] , [2] , [3] , [4] . After induction of the oncogenic KRas G12D allele, Lox-Stop-Lox-KRas G12D mice rapidly develop non-small cell lung carcinomas in a stepwise process that leads from epithelial hyperplasia to benign adenomas and malignant adenocarcinomas [23] , [27] . KRas G12D expression and simultaneous deletion of Atg5 is achieved by adenoviral delivery of Cre recombinase via inhalation (AdCre). Deletion of Atg5 in the KRas G12D -driven lung cancer model results in markedly prolonged survival; the mean survival time of KRas;Atg5 +/+ littermate controls is 144 days post AdCre infection, whereas the mean survival of KRas;Atg5 fl/fl mice is 208 days post AdCre infection. Mice carrying heterozygous mutations for Atg5 ( KRas;Atg5 fl/+ ) resemble KRas;Atg5 +/+ mice with a mean survival time of 140 days after AdCre inhalation ( Fig. 1a ). 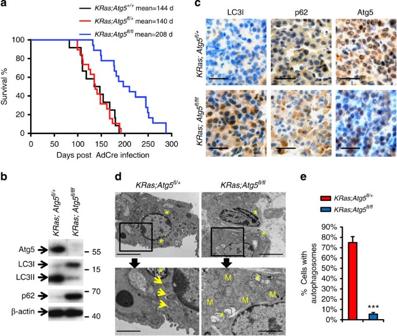Figure 1: Enhanced survival of autophagy-deficientKRas;Atg5fl/flmice. (a) The Kaplan–Meier survival curves forKRas;Atg5+/+(n=12),KRas;Atg5fl/+(n=19) andKRas;Atg5fl/fl(n=18) littermate mice injected intranasally with AdCre (2.5 × 107p.f.u.).P<0.01 (log-rank test) between theKRas;Atg5fl/flcohort and controls. (b) Western blot analysis for Atg5, LC3I and LC3II and p62 in purified primary lung tumour cells. Representative data are shown for tumour cells isolated fromKRas;Atg5fl/+andKRas;Atg5fl/flmice 18 weeks after AdCre inhalation. β-actin is shown as a loading control. (c) Immunohistochemistry to detect LC3I, p62 and Atg5 in tumours fromKRas;Atg5fl/+andKRas;Atg5fl/flmice 18 weeks after AdCre inhalation. Note highly elevated levels of LC3I and p62, both indicative of defective autophagy, inKRas;Atg5fl/fltumours. Scale bars, 50 μm. (d,e) Impaired formation of autophagosomes (arrows) inKRas;Atg5fl/fltumour cells. (d) Representative electron microscopy images are shown forKRas;Atg5fl/+andKRas;Atg5fl/fltumours 18 weeks after AdCre inhalation. Scale bars, 5 μm for upper and 2 μm for lower panels. M, mitochondria; *, lamellar bodies (Corpuscula lamellariae), rare cell organelles containing surfactant lipoproteins characteristic for type II pneumocytes. (e) Mean percentages (±s.e.m.) of tumour cells with detectable autophagosomes or autolysosomes, counted on electron microscopy images.n>=8 mice per genotype and at least 20 intact cells for each electron microscopy section were counted. ***P<0.001 (χ2-test of a generalized linear model with logit link assessing the genotype effect). Figure 1: Enhanced survival of autophagy-deficient KRas;Atg5 fl/fl mice. ( a ) The Kaplan–Meier survival curves for KRas;Atg5 +/+ ( n =12), KRas;Atg5 fl/+ ( n =19) and KRas;Atg5 fl/fl ( n =18) littermate mice injected intranasally with AdCre (2.5 × 10 7 p.f.u.). P <0.01 (log-rank test) between the KRas;Atg5 fl/fl cohort and controls. ( b ) Western blot analysis for Atg5, LC3I and LC3II and p62 in purified primary lung tumour cells. Representative data are shown for tumour cells isolated from KRas;Atg5 fl/+ and KRas;Atg5 fl/fl mice 18 weeks after AdCre inhalation. β-actin is shown as a loading control. ( c ) Immunohistochemistry to detect LC3I, p62 and Atg5 in tumours from KRas;Atg5 fl/+ and KRas;Atg5 fl/fl mice 18 weeks after AdCre inhalation. Note highly elevated levels of LC3I and p62, both indicative of defective autophagy, in KRas;Atg5 fl/fl tumours. Scale bars, 50 μm. ( d , e ) Impaired formation of autophagosomes (arrows) in KRas;Atg5 fl/fl tumour cells. ( d ) Representative electron microscopy images are shown for KRas;Atg5 fl/+ and KRas;Atg5 fl/fl tumours 18 weeks after AdCre inhalation. Scale bars, 5 μm for upper and 2 μm for lower panels. M, mitochondria; *, lamellar bodies ( Corpuscula lamellariae ), rare cell organelles containing surfactant lipoproteins characteristic for type II pneumocytes. ( e ) Mean percentages (±s.e.m.) of tumour cells with detectable autophagosomes or autolysosomes, counted on electron microscopy images. n >=8 mice per genotype and at least 20 intact cells for each electron microscopy section were counted. *** P <0.001 ( χ 2 -test of a generalized linear model with logit link assessing the genotype effect). Full size image Atg5 -deficient lung tumours show efficient deletion of Atg5 protein and impaired autophagy as determined by enhanced expression of p62/SQSTM1, reduction in LC3 lipidation ( Fig. 1b,c , Supplementary Fig. S13 and markedly reduced formation of autophagosomes and autolysosomes detectable by electron microscopy ( Fig. 1d,e ; Fig. 2a ). In the lung tumour cells from KRas;Atg5 fl/fl mice, we detect increased numbers of swollen mitochondria ( Fig. 2b ) with scarce or disordered cristae ( Fig. 2c ), indicative of impaired mitophagy. In line with these ultrastructural alterations and despite the increased mitochondrial mass, oxidative phosphorylation and ATP production are significantly impaired in isolated lung tumour cells from KRas;Atg5 fl/fl mice at 6 weeks ( Fig. 2d,e ) and 18 weeks ( Fig. 2f,g ) after AdCre inhalation, as assessed by Seahorse profiling. The differences in mitochondrial bioenergetics are more pronounced at the early stage, most probably reflecting metabolic adaptation. Gene set enrichment analysis (GSEA) further revealed that gene sets related to mitochondrial function are significantly enriched in KRas;Atg5 fl/+ compared with KRas;Atg5 fl/fl lung tumours ( Supplementary Fig. S1a,b ). Thus, we have generated mice with a specific defect in Atg5 -dependent autophagy in KRas G12D -driven lung cancer cells. Disabled autophagy results in markedly impaired mitophagy and altered energy homeostasis of tumour cells and, importantly, prolonged survival of lung cancer-bearing mice. 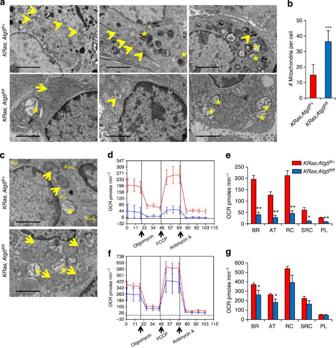Figure 2: Impaired mitophagy and bioenergetics inAtg5-deficient,KRasG12D-driven lung tumour cells. (a) Representative electron microscopy images of autolysosomes (left panels), autophagosomes (middle panels) and mitophagy (right panels), all indicated by arrows, in lung tumour cells from controlKRas;Atg5fl/+mice 18 weeks after AdCre inhalation. Note the near-to-complete absence of such structures in the lung tumour cells fromKRas;Atg5fl/fllittermates. Very rarely, we found cells with one autolysosome (left panels) or one single autophagosome (middle panels; arrows) inKRas;Atg5fl/fltumours, whereas such structures can frequently be seen within singleKRas;Atg5fl/+tumour cells. Of note, the presence of a single autophagosome or a single autolysosome was scored as a positive event inFig. 1e. Also note aberrant mitochondrial morphologies and increased mitochondrial numbers inKRas;Atg5fl/fltumour cells. * indicates lamellar bodies. Scale bars, 2 μm. (b) Mean numbers (±s.e.m.) of mitochondria per lung tumour cell fromKRas;Atg5fl/+andKRas;Atg5fl/flmice 18 weeks after tumour induction. Numbers of mitochondria were determined by electron microscopy.n≥8 mice per genotype and a minimum of 20 intact cells were counted per sample. ***P<0.001 (χ2-test assessing the genotype effect in a generalized linear model with log link). (c) Mitochondria (arrows) inKRas;Atg5fl/+andKRas;Atg5fl/fllung tumour cells 18 weeks after AdCre inhalation. Note markedly altered mitochondrial morphology, that is, disorganized matrix structures, rounding and enlargement in the autophagy-defectiveKRas;Atg5fl/flcells. Au, autophagosomes; Au-L, autolysosome; *, lamellar bodies. Scale bars, 2 μm. (d–g) Bioenergetics profiling of purified tumour cells fromKRas;Atg5fl/+andKRas;Atg5fl/flmice (e) 6 weeks and (g) 18 weeks after tumour induction. Representative experimental data are shown. Oxygen consumption rates (OCR) were used to detect the bioenergetics profiles of purified tumour cells using a Seahorse Bioscience 24XF extracellular flux analyser. OCR±s.e.m. were recorded to construct bioenergetics profiles for basal respiration (BR), ATP turnover (AT), respiratory capacity (RC), spare respiratory capacity (SRC) and proton leakage (PL). A minimum of seven different samples were analysed for each group. *P<0.05; **P<0.01(unpaired, two-sidedt-test). Figure 2: Impaired mitophagy and bioenergetics in Atg5 -deficient, KRas G12D -driven lung tumour cells. ( a ) Representative electron microscopy images of autolysosomes (left panels), autophagosomes (middle panels) and mitophagy (right panels), all indicated by arrows, in lung tumour cells from control KRas;Atg5 fl/+ mice 18 weeks after AdCre inhalation. Note the near-to-complete absence of such structures in the lung tumour cells from KRas;Atg5 fl/fl littermates. Very rarely, we found cells with one autolysosome (left panels) or one single autophagosome (middle panels; arrows) in KRas;Atg5 fl/fl tumours, whereas such structures can frequently be seen within single KRas;Atg5 fl/+ tumour cells. Of note, the presence of a single autophagosome or a single autolysosome was scored as a positive event in Fig. 1e . Also note aberrant mitochondrial morphologies and increased mitochondrial numbers in KRas;Atg5 fl/fl tumour cells. * indicates lamellar bodies. Scale bars, 2 μm. ( b ) Mean numbers (±s.e.m.) of mitochondria per lung tumour cell from KRas;Atg5 fl/+ and KRas;Atg5 fl/fl mice 18 weeks after tumour induction. Numbers of mitochondria were determined by electron microscopy. n ≥8 mice per genotype and a minimum of 20 intact cells were counted per sample. *** P <0.001 ( χ 2 -test assessing the genotype effect in a generalized linear model with log link). ( c ) Mitochondria (arrows) in KRas;Atg5 fl/+ and KRas;Atg5 fl/fl lung tumour cells 18 weeks after AdCre inhalation. Note markedly altered mitochondrial morphology, that is, disorganized matrix structures, rounding and enlargement in the autophagy-defective KRas;Atg5 fl/fl cells. Au, autophagosomes; Au-L, autolysosome; *, lamellar bodies. Scale bars, 2 μm. ( d – g ) Bioenergetics profiling of purified tumour cells from KRas;Atg5 fl/+ and KRas;Atg5 fl/fl mice ( e ) 6 weeks and ( g ) 18 weeks after tumour induction. Representative experimental data are shown. Oxygen consumption rates (OCR) were used to detect the bioenergetics profiles of purified tumour cells using a Seahorse Bioscience 24XF extracellular flux analyser. OCR±s.e.m. were recorded to construct bioenergetics profiles for basal respiration (BR), ATP turnover (AT), respiratory capacity (RC), spare respiratory capacity (SRC) and proton leakage (PL). A minimum of seven different samples were analysed for each group. * P <0.05; ** P <0.01(unpaired, two-sided t -test). Full size image Enhanced tumour initiation Intriguingly, although KRas;Atg5 fl/fl animals exhibit overall prolonged survival, we observe enhanced numbers of hyperplastic tumour foci as early as 2 weeks after AdCre inhalation ( Fig. 3a,b ). Six weeks after AdCre administration, the tumour burden in KRas;Atg5 fl/fl mice is significantly higher than that in KRas;Atg5 fl/+ controls ( Fig. 3c ; Supplementary Fig. S2a ). Eight weeks after AdCre challenge, we observe a similar tumour burden and at 12 weeks tumours from KRas;Atg5 fl/fl mice exhibited significantly reduced growth as compared with Atg5-expressing KRas;Atg5 fl/+ littermates ( Fig. 3c ; Supplementary Fig. S2b ). Reduced overall tumour burden is also observed at 18 weeks after AdCre inhalation ( Fig. 3c,d ; Supplementary Fig. S2c ). Statistical analysis using logistic growth, Malthusian parameters or cumulative link mixed effects (R-clmm) modelling confirm initially increased growth rates and delayed lung tumour progression in KRas;Atg5 fl/fl mice ( Supplementary Fig. S3a,b ). 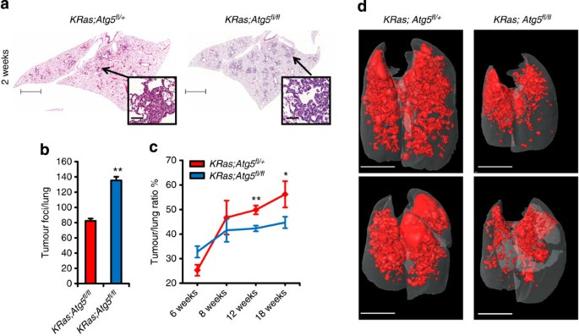Figure 3: Elevated tumour initiation and delayed tumour progression. (a) Increased tumour initiation inKRas;Atg5fl/flmice as compared withKRas;Atg5fl/+littermates. Representative histological sections at 2 weeks after AdCre inhalation are shown. Insets show typical lung lesions. Haematoxylin and eosin staining. Scale bars, 2 mm for whole lung section; 50 μm for insets. (b) Quantification of numbers of hyperplastic lesions/per lung (mean values±s.e.m.) inKRas;Atg5fl/+andKRas;Atg5fl/flmice 2 weeks after AdCre inhalation.n=6 per group. **P<0.01 (χ2-test assessing the genotype effect in a generalized linear model with log link). (c) Tumour growth curves based on mean tumour-to-lung area ratios (±s.e.m.) determined inKRas;Atg5fl/+andKRas;Atg5fl/fllittermates at the indicated time points. At least three different planes from each lung were analysed.n≥6 per cohort for each time point. *P<0.05, **P<0.01 (unpaired, two-sided Wicoxon test). (d) MicroCT analysis of lung tumours ofKRas;Atg5fl/+andKRas;Atg5fl/fllittermate mice 18 weeks after AdCre inhalation. Representative data from individual mice are shown. Scale bars, 5 mm. Figure 3: Elevated tumour initiation and delayed tumour progression. ( a ) Increased tumour initiation in KRas;Atg5 fl/fl mice as compared with KRas;Atg5 fl/+ littermates. Representative histological sections at 2 weeks after AdCre inhalation are shown. Insets show typical lung lesions. Haematoxylin and eosin staining. Scale bars, 2 mm for whole lung section; 50 μm for insets. ( b ) Quantification of numbers of hyperplastic lesions/per lung (mean values±s.e.m.) in KRas;Atg5 fl/+ and KRas;Atg5 fl/fl mice 2 weeks after AdCre inhalation. n =6 per group. ** P <0.01 ( χ 2 -test assessing the genotype effect in a generalized linear model with log link). ( c ) Tumour growth curves based on mean tumour-to-lung area ratios (±s.e.m.) determined in KRas;Atg5 fl/+ and KRas;Atg5 fl/fl littermates at the indicated time points. At least three different planes from each lung were analysed. n ≥6 per cohort for each time point. * P <0.05, ** P <0.01 (unpaired, two-sided Wicoxon test). ( d ) MicroCT analysis of lung tumours of KRas;Atg5 fl/+ and KRas;Atg5 fl/fl littermate mice 18 weeks after AdCre inhalation. Representative data from individual mice are shown. Scale bars, 5 mm. Full size image We next graded the malignant progression of lung tumours using established histopathological criteria [28] . Two weeks after AdCre inhalation, we only observe hyperplasias, irrespective of the status of Atg5. At 6 weeks, adenomas become detectable in a small fraction of the lung tumours and this progression to the adenoma stage is significantly more frequent in KRas;Atg5 fl/fl animals ( Fig. 4a,b ). Interestingly, proliferation of lung tumours in KRas;Atg5 fl/fl mice, as detected by Ki67 staining, is comparable to that of control littermates 6 weeks after AdCre inhalation ( Supplementary Fig. S4a ). In line with previous studies [29] , [30] , we fail to detect apoptotic cells in KRas G12D -induced lung lesions from littermate control or KRas;Atg5 fl/fl mice at this time point. 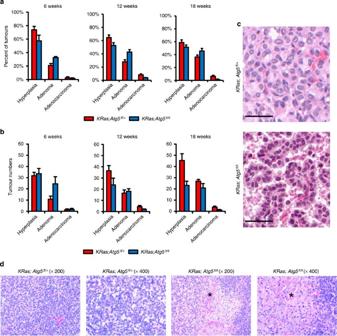Figure 4: Tumour progression. (a) Distribution and (b) absolute numbers of hyperplastic lesions, adenomas and adenocarcinomas inKRas;Atg5fl/+andKRas;Atg5fl/fllittermate mice 6, 12 and 18 weeks post AdCre infection. Data are shown as means±s.e.m.;n=6 per group. Combining the tumour progression data from 6, 12 and 18 weeks, a cumulative linked mixed model (clmm) analysis showed also a significant dependency of tumour progression on the genotype;P<0.05 (χ2-test of clmms assessing the genotype effect). Applying generalized linear-mixed effects (glmer) models with logit link to individual time points, shows a significant dependency of the transition from hyperplastic lesions to adenomas (12 weeks,P<0.05) and from adenomas to adenocarcinomas (12 weeks,P<0.01 and 18 weeks,P<0.01) on the mouse genotype (the last threeP-values are fromχ2-tests of a generalized linear models with logit link assessing the genotype effect). (c,d) Histological analyses (haematoxylin and eosin staining) of lung tumours inKRas;Atg5fl/+andKRas;Atg5fl/fllittermates 18 weeks after AdCre inhalation. (c) Nuclear and cellular polymorphy, more dense and sometimes irregular chromatin as well as more nucleoli in tumour cells ofKRas;Atg5fl/+mice as compared withKRas;Atg5fl/fltumours. Sections were analysed 18 weeks after AdCre inhalation. Scale bars, 50 μm. (d)KRas;Atg5fl/fltumours exhibited markedly increased apoptotic figures and necrotic areas in the centre of larger tumours (asterisk). Figure 4: Tumour progression. ( a ) Distribution and ( b ) absolute numbers of hyperplastic lesions, adenomas and adenocarcinomas in KRas;Atg5 fl/+ and KRas;Atg5 fl/fl littermate mice 6, 12 and 18 weeks post AdCre infection. Data are shown as means±s.e.m. ; n =6 per group. Combining the tumour progression data from 6, 12 and 18 weeks, a cumulative linked mixed model (clmm) analysis showed also a significant dependency of tumour progression on the genotype; P <0.05 ( χ 2 -test of clmms assessing the genotype effect). Applying generalized linear-mixed effects (glmer) models with logit link to individual time points, shows a significant dependency of the transition from hyperplastic lesions to adenomas (12 weeks, P <0.05) and from adenomas to adenocarcinomas (12 weeks, P <0.01 and 18 weeks, P <0.01) on the mouse genotype (the last three P -values are from χ 2 -tests of a generalized linear models with logit link assessing the genotype effect). ( c , d ) Histological analyses (haematoxylin and eosin staining) of lung tumours in KRas;Atg5 fl/+ and KRas;Atg5 fl/fl littermates 18 weeks after AdCre inhalation. ( c ) Nuclear and cellular polymorphy, more dense and sometimes irregular chromatin as well as more nucleoli in tumour cells of KRas;Atg5 fl/+ mice as compared with KRas;Atg5 fl/fl tumours. Sections were analysed 18 weeks after AdCre inhalation. Scale bars, 50 μm. ( d ) KRas;Atg5 fl/fl tumours exhibited markedly increased apoptotic figures and necrotic areas in the centre of larger tumours (asterisk). Full size image At 12 and 18 weeks after AdCre inhalation, we observe comparable numbers of hyperplastic lesions; however, progression to lung adenocarcinomas is markedly impaired in KRas;Atg5 fl/fl mice ( Fig. 4a,b ); pathological assessment reveals increased signs of malignancy (mitotic figures, cellular and nuclear polymorphy) in KRas;Atg5 fl/+ control tumours, whereas KRas;Atg5 fl/fl tumours are composed by oncocytes, that is, cells with a large eosinophilic cytoplasm and relatively small round nuclei ( Fig. 4c ). These autophagy-deficient tumours exhibit markedly increased apoptotic figures and, especially in the centre of larger tumours, the development of necrotic areas ( Fig. 4d ). In situ immunohistochemistry further shows that proliferation of lung tumour cells was markedly impaired in the KRas;Atg5 fl/fl mice ( Supplementary Fig. S4b ). Moreover, we observe increased senescence as detected by promyelocytic leukemia (PML) immunostaining ( Supplementary Fig. S4c ) as a marker for cellular aging [31] . Immunoblotting further reveals increased amounts of cleaved active caspases-3 and -8 ( Supplementary Fig. S5a ). In situ detection of active caspase-3 as well as terminal deoxynucleotidyl transferase dUTP nick-end labelling staining confirms enhanced death of KRas;Atg5 fl/fl lung tumour cells ( Supplementary Fig. S5b ). Thus, loss of Atg5-regulated autophagy accelerates oncogenic transformation in the KRas G12D -driven lung cancer model, initially increasing tumour burden. However, autophagy-deficient adenomas subsequently exhibit reduced malignant progression to adenocarcinomas, resulting in impaired proliferation and enhanced death of tumour cells, as well as in a marked survival advantage of lung tumour-bearing mice. Gene expression profiling How can we explain the paradoxical increase in tumour initiation, but improved overall survival of mice bearing Atg5-deficient tumours? We first profiled gene expression in lung tumours isolated from control and KRas;Atg5 fl/fl littermates at 18 weeks after AdCre inhalation. Functional enrichment analyses (Ingenuity) and GSEA [32] reveals that genes annotated to inflammation are markedly upregulated in lung tumours from KRas;Atg5 fl/fl mice as compared with KRas;Atg5 fl/+ animals ( Supplementary Fig. S6a,b ). Upregulation of defined inflammatory genes is confirmed by quantitative PCR ( Supplementary Fig. S6c ). The most induced gene is Cxcl5 , a chemokine that regulates the formation of new tumour vasculature [33] . Upregulation of Cxcl5 is confirmed by enzyme-linked immunosorbent assay (ELISA; Supplementary Fig. S7a ) and increased neo-angiogenesis in the lungs from KRas;Atg5 fl/fl mice is corroborated by immunostaining for Von Willebrand factor ( Supplementary Fig. S7b ). Consistent with the upregulation of pro-inflammatory genes, we observe marked infiltration of KRas;Atg5 fl/fl tumours by F4/80 + macrophages ( Supplementary Fig. S7c ). Besides genes linked to inflammation, we also observe marked and concerted upregulation of genes annotated to glutathione metabolism and oxidative stress ( Supplementary Fig. S6a,b,d ). To corroborate these findings, we performed gene expression analyses on primary pneumocytes isolated from KRas;Atg5 fl/+ and KRas;Atg5 fl/fl littermates rather than transformed cells from established tumours using Ilumina messenger RNA sequencing (mRNAseq). Pneumocytes are cultured for 6 days and infected with AdCre to induce expression of the KRas G12D oncogene and concomitant Atg5 deletion ( Fig. 5a,b ). Genes differentially expressed between KRas;Atg5 fl/fl and control KRas;Atg5 fl/+ pneumocytes are selected using DESeq. Gene ontology (GO) terms show enrichment of genes annotated for locomotion and leukocyte migration, cell adhesion, blood vessel remodelling, immune responses, oxidative stress or hypoxia in KRas;Atg5 fl/fl as compared with control KRas;Atg5 fl/+ pneumocytes ( Fig. 5c ). Ingenuity pathway analysis (IPA) confirms that genes involved in ‘cellular movement’, ‘immune cell trafficking’, ‘inflammatory response’, ‘cell death and survival’, ‘free radical scavenging’, ‘metabolism of reactive oxygen species (ROS)’ and ‘oxidative stress response’ are overrepresented in KRas;Atg5 fl/fl pneumocytes ( Fig. 6a ). Typical examples for gene expression changes for genes involved in inflammation ( il1β ) and the oxidative stress response ( nrf2 , nqo1 ) are shown in Supplementary Fig. S8 . Altogether, our data reveal that, in established tumours as well as temporally controlled deletion experiments in primary pneumocytes, impaired autophagy results in a marked induction of gene annotated to inflammation, angiogenesis, hypoxia and the oxidative stress response. 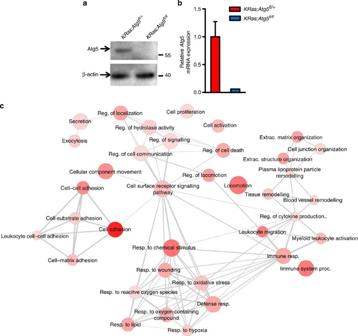Figure 5: Gene expression networks in primary pneumocytes. (a,b) Induction ofAtg5deletion in pneumocytes isolated fromKRas;Atg5fl/+andKRas;Atg5fl/flmice. (a) Primary pneumocytes were infected with AdCre for 96 h and Atg5 protein expression determined by western blot. β-actin is shown as a loading control. (b) Atg5 mRNA expression was determined by quantitative PCR. Data are shown as mean relative mRNA expression±s.e.m. inKRas;Atg5fl/fltumours as compared with tumours fromKRas;Atg5fl/+mice (set to 1). Values were normalized to β-actin mRNA expression.n=3 per group. (c) GO terms showed enrichment of genes annotated for locomotion and leukocyte migration, cell adhesion, blood vessel remodelling, immune responses, oxidative stress or hypoxia inKRas;Atg5fl/flas compared with controlKRas;Atg5fl/+pneumocytes. Enrichment and vizualization analysis was performed using GOrilla and REViGO, with colour depth indicating the enrichment significance (P-value). Differentially expressed genes betweenKRas;Atg5fl/flandKRas;Atg5fl/+pneumocytes were selected using DESeq (‘blind’ variance estimation, fold-change>2, adjP<0.05, false discovery rate adjusted for multiple testing). Figure 5: Gene expression networks in primary pneumocytes. ( a , b ) Induction of Atg5 deletion in pneumocytes isolated from KRas;Atg5 fl/+ and KRas;Atg5 fl/fl mice. ( a ) Primary pneumocytes were infected with AdCre for 96 h and Atg5 protein expression determined by western blot. β-actin is shown as a loading control. ( b ) Atg5 mRNA expression was determined by quantitative PCR. Data are shown as mean relative mRNA expression±s.e.m. in KRas;Atg5 fl/fl tumours as compared with tumours from KRas;Atg5 fl/+ mice (set to 1). Values were normalized to β-actin mRNA expression. n =3 per group. ( c ) GO terms showed enrichment of genes annotated for locomotion and leukocyte migration, cell adhesion, blood vessel remodelling, immune responses, oxidative stress or hypoxia in KRas;Atg5 fl/fl as compared with control KRas;Atg5 fl/+ pneumocytes. Enrichment and vizualization analysis was performed using GOrilla and REViGO, with colour depth indicating the enrichment significance ( P -value). Differentially expressed genes between KRas;Atg5 fl/fl and KRas;Atg5 fl/+ pneumocytes were selected using DESeq (‘blind’ variance estimation, fold-change>2, adj P <0.05, false discovery rate adjusted for multiple testing). 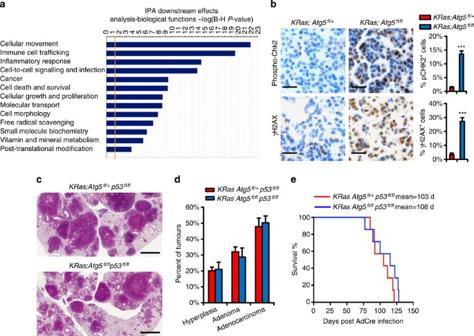Figure 6: P53 controls progression ofAtg5-deficient KRasG12D-driven tumour. (a) Ingenuity analysis of genes differentially expressed betweenKRas;Atg5fl/+andKRas;Atg5fl/flpneumocytes determined by RNAseq (set selection using DESeq with adjP<0.05, fold-change>2 cutoffs). Biological functions overrepresented in the differentially expressed gene sets are shown with the respective Bonferroni–HochbergP-value indicating enrichment significance. (b) Representative immunohistochemistry and quantitative assessment of γH2AX and phospho-Chk2 in lung tumours fromKRas;Atg5fl/+andKRas;Atg5fl/fllittermates 18 weeks after AdCre inhalation. For γH2AX and phospho-Chk2 staining, sections were scored independently in a double-blinded manner. Data are shown as mean percentages (±s.e.m.) of positive cells per total cell numbers.n=6 mice per genotype. Scale bars, 50 μm. ***P<0.001 (χ2-test of a generalized linear model with logit link assessing the genotype effect). (c) Representative histological lung sections ofKRas;Atg5fl/+;p53fl/flandKRas;Atg5fl/fl;p53fl/fllittermate mice 16 weeks after AdCre inhalation. Scale bars, 2 mm. (d) Distribution of hyperplastic lesions, adenomas and adenocarcinomas (±s.e.m.) inKRas;Atg5fl/+;p53fl/flandKRas;Atg5fl/fl;p53fl/fllittermates 16 weeks post AdCre infection (n=4 per genotype). (e) The Kaplan–Meier survival curves forKRas;Atg5fl/+;p53fl/fl(n=8) andKRas;Atg5fl/fl;p53fl/fl(n=9) littermate mice injected intranasally with AdCre (2.5 × 107p.f.u.). There was no statistical difference between the cohorts (log-rank test). Full size image Figure 6: P53 controls progression of Atg5 -deficient KRas G12D -driven tumour. ( a ) Ingenuity analysis of genes differentially expressed between KRas;Atg5 fl/+ and KRas;Atg5 fl/fl pneumocytes determined by RNAseq (set selection using DESeq with adj P <0.05, fold-change>2 cutoffs). Biological functions overrepresented in the differentially expressed gene sets are shown with the respective Bonferroni–Hochberg P -value indicating enrichment significance. ( b ) Representative immunohistochemistry and quantitative assessment of γH2AX and phospho-Chk2 in lung tumours from KRas;Atg5 fl/+ and KRas;Atg5 fl/fl littermates 18 weeks after AdCre inhalation. For γH2AX and phospho-Chk2 staining, sections were scored independently in a double-blinded manner. Data are shown as mean percentages (±s.e.m.) of positive cells per total cell numbers. n =6 mice per genotype. Scale bars, 50 μm. *** P <0.001 ( χ 2 -test of a generalized linear model with logit link assessing the genotype effect). ( c ) Representative histological lung sections of KRas;Atg5 fl/+ ;p53 fl/fl and KRas;Atg5 fl/fl ;p53 fl/fl littermate mice 16 weeks after AdCre inhalation. Scale bars, 2 mm. ( d ) Distribution of hyperplastic lesions, adenomas and adenocarcinomas (±s.e.m.) in KRas;Atg5 fl/+ ;p53 fl/fl and KRas;Atg5 fl/fl ;p53 fl/fl littermates 16 weeks post AdCre infection ( n =4 per genotype). ( e ) The Kaplan–Meier survival curves for KRas;Atg5 fl/+ ;p53 fl/fl ( n =8) and KRas;Atg5 fl/fl ;p53 fl/fl ( n =9) littermate mice injected intranasally with AdCre (2.5 × 10 7 p.f.u.). There was no statistical difference between the cohorts (log-rank test). Full size image P53 has a role in tumour progression In line with enhanced metabolic stress, increased phosphorylation of histone H2AX (γH2AX) indicates an exacerbated DNA damage response in lung tumours of KRas;Atg5 fl/fl mice 6 weeks after AdCre inhalation relative to KRas;Atg5 fl/+ control tumours ( Supplementary Fig. S9a ). γH2AX-positive cells are not visible in adjacent normal pneumocytes. Immunostaining for phospho-Chk2 confirming an increased DNA damage response linked to deficient autophagy ( Supplementary Fig. S9b ). In late-stage autophagy-defective tumours, we again detect markedly increased γ-H2AX and phospho-Chk2 ( Fig. 6b ). This is of particular interest since recent studies have shown that the DNA damage response can be activated by oncogenic stress in early tumour lesions and constitutes an anticancer barrier by activating the p53 pathway [34] . In addition to the DNA damage response, oxidative stress might also contribute to p53 activation [35] . We therefore speculated that the p53 tumour suppressor pathway might induce a brake in the malignant progression of autophagy-defective lung tumours. To provide direct evidence that p53 is indeed functionally relevant for the impaired tumour progression and enhanced survival of KRas;Atg5 fl/fl mice, we introduced a p53 floxed allele generating KRas;Atg5 fl/fl ; p53 fl/fl and KRas;Atg5 fl/+ ;p53 fl/fl littermate mice. Loss of p53 in KRas;Atg5 fl/fl animals results in markedly accelerated lung cancer progression and the development of adenocarcinomas resembling those from autophagy-competent KRas;Atg5 fl/+ tumours ( Fig. 6c,d ; Supplementary Fig. S10a ). Pathological assessment reveals marked signs of malignancy including mitotic figures, cellular and nuclear pleomorphism, as well as local invasion in both KRas;Atg5 fl/+ ;p53 fl/fl and KRas;Atg5 fl/fl ; p53 fl/fl tumours ( Supplementary Fig. S10b ). Importantly, tumour cell-specific deletion of p53 completely abolishes the overall survival advantage of KRas;Atg5 fl/fl mice ( Fig. 6e ). p53 deficiency also abrogated the differences in tumour initiation at 2 weeks after AdCre inhalation ( Supplementary Fig. S10c ). Moreover, the loss of p53 in both KRas;Atg5 fl/+ and KRas;Atg5 fl/fl tumours results in a major increase in cells with γH2AX + DNA damage foci, both in early hyperplastic lesions and in late-stage lung cancers ( Supplementary Fig. S10d ). Although additional mechanisms cannot be excluded, these results indicate that the p53 tumour suppressor pathway is a critical brake that regulates the progression from adenoma to adenocarcinoma in autophagy-deficient lung tumours. Autophagy couples to early immunosurveillance Whereas p53 clearly controls the overall survival and progression from adenomas to carcinomas in autophagy-deficient tumours, removal of p53 does not affect the initial increase in the number of tumour foci found in the context of disabled autophagy. Driven by the considerations that immunosurveillance mechanisms determine the onset of oncogenesis much more than final tumour progression [36] and that autophagy can provide signals to activate the immune system [37] , [38] , we performed comparative immunoprofiling of the early pulmonary lesions from KRas;Atg5 fl/fl and KRas;Atg5 fl/+ mice. When we monitor tumour-infiltrating cells at 6 weeks after AdCre challenge, we observed comparable numbers of CD3ε + T cells in both control and KRas;Atg5 fl/fl littermates ( Fig. 7a ). Intriguingly, although the total number of infiltrating T cells is comparable, the numbers of intratumoral FoxP3 + regulatory T cells (Tregs), known to suppress the immune system [39] , [40] , [41] , are markedly increased in KRas;Atg5 fl/fl mice ( Fig. 7b ). 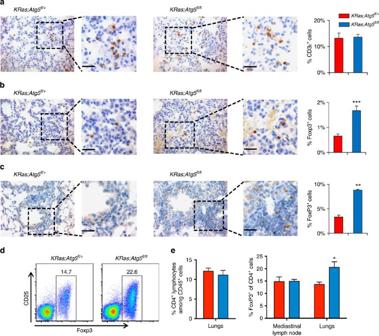Figure 7: Accumulation of Tregs in lungs of mice with early autophagy-deficient hyperplastic lesions. (a,b) Representative immunohistochemistry and quantitative assessment of (a) tumour-infiltrating CD3ε-positive T cells and (b) FoxP3+Tregs in lung tumours fromKRas;Atg5fl/+andKRas;Atg5fl/fllittermates 6 weeks after AdCre inhalation. Data are shown as mean percentages (±s.e.m.) of the indicated cell types per total cell numbers in the tumour areas. Only cells within tumours were scored. At least six mice per genotype were analysed. Scale bars, 50 μm. ***P<0.001(χ2-test assessing the genotype effect in a generalized linear model with logit link). (c) Representative immunohistochemistry and quantitative assessment of FoxP3+Tregs in lung tumours fromKRas;Atg5fl/+andKRas;Atg5fl/fllittermates 2 weeks after AdCre inhalation. Data are shown as mean percentages (±s.e.m.) of FoxP3+cells among total cell numbers in the tumour areas. Only cells within tumours were scored. At least six mice per genotype were analysed. Scale bars, 50 μm. **P<0.01(χ2-test assessing the genotype effect in a generalized linear model with logit link). (d) FACS blots to detect CD25+FoxP3+Treg cells in lungs 2 weeks after AdCre inhalation. Cells were gated on CD4+populations. Numbers indicate percentages among total CD4+cells in the lungs. (e) Mediastinal lymph node and lung cells were isolated fromKRas;Atg5fl/+andKRas;Atg5fl/fllittermates 2 weeks after AdCre inhalation and stained for flow cytometric analysis as described in Methods. The left panel shows the percentage of CD4+T cells among all lung-infiltrating CD45+haematopoietic cells (±s.e.m.). The right panel shows the percentage of FoxP3+cells among CD4+T cells in mediastinal lymph nodes and lungs (±s.e.m.).n=4 per genotype; *P<0.05 (unpaired, two-sidedt-test). Figure 7: Accumulation of Tregs in lungs of mice with early autophagy-deficient hyperplastic lesions. ( a , b ) Representative immunohistochemistry and quantitative assessment of ( a ) tumour-infiltrating CD3ε-positive T cells and ( b ) FoxP3 + Tregs in lung tumours from KRas;Atg5 fl/+ and KRas;Atg5 fl/fl littermates 6 weeks after AdCre inhalation. Data are shown as mean percentages (±s.e.m.) of the indicated cell types per total cell numbers in the tumour areas. Only cells within tumours were scored. At least six mice per genotype were analysed. Scale bars, 50 μm. *** P <0.001( χ 2 -test assessing the genotype effect in a generalized linear model with logit link). ( c ) Representative immunohistochemistry and quantitative assessment of FoxP3 + Tregs in lung tumours from KRas;Atg5 fl/+ and KRas;Atg5 fl/fl littermates 2 weeks after AdCre inhalation. Data are shown as mean percentages (±s.e.m.) of FoxP3 + cells among total cell numbers in the tumour areas. Only cells within tumours were scored. At least six mice per genotype were analysed. Scale bars, 50 μm. ** P <0.01( χ 2 -test assessing the genotype effect in a generalized linear model with logit link). ( d ) FACS blots to detect CD25 + FoxP3 + Treg cells in lungs 2 weeks after AdCre inhalation. Cells were gated on CD4 + populations. Numbers indicate percentages among total CD4 + cells in the lungs. ( e ) Mediastinal lymph node and lung cells were isolated from KRas;Atg5 fl/+ and KRas;Atg5 fl/fl littermates 2 weeks after AdCre inhalation and stained for flow cytometric analysis as described in Methods. The left panel shows the percentage of CD4 + T cells among all lung-infiltrating CD45 + haematopoietic cells (±s.e.m.). The right panel shows the percentage of FoxP3 + cells among CD4 + T cells in mediastinal lymph nodes and lungs (±s.e.m.). n =4 per genotype; * P <0.05 (unpaired, two-sided t -test). Full size image To expand these studies to initial steps of transformation, we analysed pulmonary immune cells 2 weeks after AdCre inhalation, that is, when the first hyperplastic lesions have formed. We again observe increased numbers of CD25 + FoxP3 + T cells in early hyperplastic lung lesions from KRas;Atg5 fl/fl mice ( Fig. 7c ), indicating that defective autophagy causes Tregs to accumulate in developing tumours. Elevated numbers of Tregs in the lungs, but not in the local draining mediastinal lymph nodes are also seen using fluorescence activated cell sorting (FACS) analysis ( Fig. 7d,e ). No differences in the number of CD4 + TCRαβ + T cells, CD8 + TCRαβ + T cells, TCRγδ + T cells, NK cells, neutrophils and CD11b + , CD11b − or CD11c + dendritic cells can be detected between KRas;Atg5 fl/fl and control KRas;Atg5 fl/+ tumours. Moreover, expression of Helios, ICOS, LAP and PD1 on Tregs are comparable among lung and draining lymph node Tregs from both KRas;Atg5 fl/fl and control KRas;Atg5 fl/+ littermates 2 weeks after AdCre exposure. However, we detect expanded Treg numbers in lung tumours from KRas;Atg5 fl/fl mice up to 18 weeks after AdCre inhalation ( Supplementary Fig. S11 ). These data indicate that tumour-specific loss of Atg5 favours local infiltration by Tregs. To provide direct evidence that Tregs are responsible for enhanced tumour initiation in KRas;Atg5 fl/fl mice, we depleted or inhibited Tregs by means of antibodies (Abs) specific for CD25 or FR4, respectively, following previously reported protocols [42] , [43] . Depletion of Tregs using anti-CD25 Abs as well as their functional inhibition using anti-FR4 Abs revert the increased lung tumour initiation in KRas;Atg5 fl/fl mice to numbers observed in control KRas;Atg5 fl/+ mice ( Fig. 8a–d , Supplementary Fig. S12 ). Expansion of Tregs fail to occur in the lungs of Atg5 fl/fl or Atg5 fl/+ mice that do not carry the KRas mutation, thereby excluding the possibility that the Treg expansion observed in KRas;Atg5 fl/fl mice constitutes an inflammatory response to the AdCre virus challenge. Thus, defective autophagy in pneumocytes expressing an active KRas oncogene appears to trigger local expansion of Tregs that control lung tumour initiation, linking deregulated autophagy to Treg-controlled anticancer immunity. 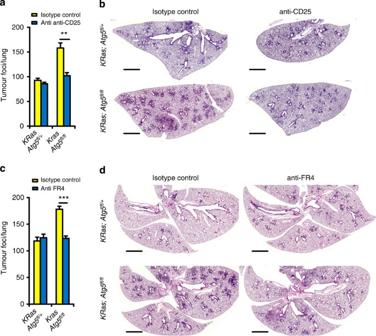Figure 8: Impaired autophagy links to immunosurveillance and enhanced lung tumour initiation. (a) Quantification of numbers of hyperplastic lesions/per lung (mean values±s.e.m.) inKRas;Atg5fl/+andKRas;Atg5fl/flmice 2 weeks after AdCre inhalation treated either with an isotype control Ab or a depleting anti-CD25 Ab.n=4 per group. **P<0.01 (χ2-test assessing the genotype effect in a generalized linear model with log link). (b) Histological lung sections ofKRas;Atg5fl/+andKRas;Atg5fl/fllittermate mice treated with an isotype control Ab or anti-CD25-immunodepleting Abs. Mice were killed 2 weeks after AdCre inhalation and their lungs were processed for histopathology. Representative lung images (haematoxylin and eosin (H&E) staining) are shown for each genotype and treatment. Scale bars, 2 mm. (c) Quantification of numbers of hyperplastic lesions/per lung (mean values±s.e.m.) inKRas;Atg5fl/+andKRas;Atg5fl/flmice 2 weeks after AdCre inhalation treated either with an isotype control Ab or an Ab specific to FR4.n=4 per group. ***P<0.001 (χ2-test assessing the genotype effect in a generalized linear model with log link). (d) Histological lung sections ofKRas;Atg5fl/+andKRas;Atg5fl/fllittermate mice treated with isotype control Abs or Abs specific to FR4. Mice were killed 2 weeks after AdCre inhalation and their lungs were processed for histopathology. Representative lung images (H&E staining) are shown for each genotype and treatment. Scale bars, 2 mm. Figure 8: Impaired autophagy links to immunosurveillance and enhanced lung tumour initiation. ( a ) Quantification of numbers of hyperplastic lesions/per lung (mean values±s.e.m.) in KRas;Atg5 fl/+ and KRas;Atg5 fl/fl mice 2 weeks after AdCre inhalation treated either with an isotype control Ab or a depleting anti-CD25 Ab. n =4 per group. ** P <0.01 ( χ 2 -test assessing the genotype effect in a generalized linear model with log link). ( b ) Histological lung sections of KRas;Atg5 fl/+ and KRas;Atg5 fl/fl littermate mice treated with an isotype control Ab or anti-CD25-immunodepleting Abs. Mice were killed 2 weeks after AdCre inhalation and their lungs were processed for histopathology. Representative lung images (haematoxylin and eosin (H&E) staining) are shown for each genotype and treatment. Scale bars, 2 mm. ( c ) Quantification of numbers of hyperplastic lesions/per lung (mean values±s.e.m.) in KRas;Atg5 fl/+ and KRas;Atg5 fl/fl mice 2 weeks after AdCre inhalation treated either with an isotype control Ab or an Ab specific to FR4. n =4 per group. *** P <0.001 ( χ 2 -test assessing the genotype effect in a generalized linear model with log link). ( d ) Histological lung sections of KRas;Atg5 fl/+ and KRas;Atg5 fl/fl littermate mice treated with isotype control Abs or Abs specific to FR4. Mice were killed 2 weeks after AdCre inhalation and their lungs were processed for histopathology. Representative lung images (H&E staining) are shown for each genotype and treatment. Scale bars, 2 mm. Full size image Adenosinergic signalling and tumour initiation In our gene expression studies we consistently find marked induction of the oxidative stress response and the hypoxia pathway. IPA indicates that hypoxia-inducible factor 1α might act as a key upstream regulator that couples to various functional pathways ( Fig. 9a ). In non-transformed autophagy-defective pneumocytes expressing oncogenic KRas as well as in tumour cells isolated 2 weeks after AdCre inhalation, we observe a marked increase in Hif1α expression ( Fig. 9b , Supplementary Fig. S13 ). One molecule regulated by Hif1α is CD39 (ref. 44 ), a plasma membrane-associated ecto-ATPase that initiates the conversion of immunostimulatory ATP into adenosine [45] . CD39 protein is indeed strongly induced in autophagy-defective, KRas-expressing cells but not in Atg5 -mutant cells that do not express oncogenic KRas ( Fig. 9c , Supplementary Fig. S13 ). CD39 induction is abrogated when hypoxia-inducible factor 1α is inhibited ( Fig. 9d , Supplementary Fig. S13 ) but not when Nrf2 or ROS production is blocked ( Fig. 9e , Supplementary Fig. S13 ). 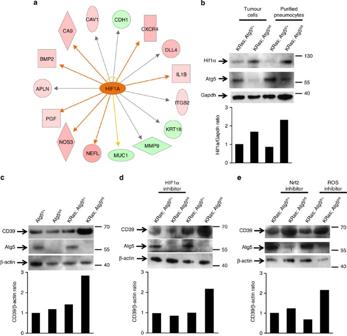Figure 9: CD39 induction in pneumocytes ofKRas;Atg5fl/flmice. (a) Ingenuity analysis identifies Hif1α as a key upstream regulator (activationz-score=2.003;P=9.43e−08) that connects to a set of upregulated (red node) or downregulated (green nodes) genes in isolatedKRas;Atg5fl/fl, non-transformed pneumocytes 48 h after infection with AdCre. Expression was determined by RNAseq. Orange edge, leads to activation; yellow edge, inconsistent state; grey edge, effect not predicted. (b) Protein expression of Hif1α, Atg5 and glyceraldehyde 3-phosphate dehydrogenase (GAPDH) in isolatedKRas;Atg5fl/+andKRas;Atg5fl/flpneumocytes (analysed at 4 days after AdCre infection) and tumours purified fromKRas;Atg5fl/+andKRas;Atg5fl/fllittermate mice at week 2 after AdCre inhalation. Quantifications of the hypoxia-inducible factor (HIF)1α/GAPDH ratios are shown for each lane; two independent blots are quantified. (c) CD39, Atg5 and as a control β-actin protein expression in isolatedAtg5fl/+, Atg5fl/fl,KRas;Atg5fl/+andKRas;Atg5fl/flpneumocytes. Protein lysated were analysed at 4 days after AdCre infections by western blot. Quantifications of the CD39/β-actin ratios are shown for each lane, normalized to theAtg5fl/+samples. Two independent blots are quantified. (d,e) CD39, Atg5 and as a control β-actin protein expression in isolatedKRas;Atg5fl/+andKRas;Atg5fl/flpneumocytes treated with the (d) HIF1α inhibitor 3-(2-(4-adamantan-1-yl-phenoxy)-acetylamino)-4-hydroxybenzoic acid methyl ester or left untreated and (e) the Nrf2 inhibitor Brusatol (100 nM) or the ROS scavengerN-acetyl-L-cysteine (5 mM). Protein lysates were analysed on day 4 by western blot. Quantifications of the CD39/β-actin ratios are shown for each lane. The inhibitors were present during the entire 4day culture period. Figure 9: CD39 induction in pneumocytes of KRas;Atg5 fl/fl mice. ( a ) Ingenuity analysis identifies Hif1α as a key upstream regulator (activation z -score=2.003; P =9.43e−08) that connects to a set of upregulated (red node) or downregulated (green nodes) genes in isolated KRas;Atg5 fl/fl , non-transformed pneumocytes 48 h after infection with AdCre. Expression was determined by RNAseq. Orange edge, leads to activation; yellow edge, inconsistent state; grey edge, effect not predicted. ( b ) Protein expression of Hif1α, Atg5 and glyceraldehyde 3-phosphate dehydrogenase (GAPDH) in isolated KRas;Atg5 fl/+ and KRas;Atg5 fl/fl pneumocytes (analysed at 4 days after AdCre infection) and tumours purified from KRas;Atg5 fl/+ and KRas;Atg5 fl/fl littermate mice at week 2 after AdCre inhalation. Quantifications of the hypoxia-inducible factor (HIF)1α/GAPDH ratios are shown for each lane; two independent blots are quantified. ( c ) CD39, Atg5 and as a control β-actin protein expression in isolated Atg5 fl/+ , Atg5 fl/fl , KRas;Atg5 fl/+ and KRas;Atg5 fl/fl pneumocytes. Protein lysated were analysed at 4 days after AdCre infections by western blot. Quantifications of the CD39/β-actin ratios are shown for each lane, normalized to the Atg5 fl/+ samples. Two independent blots are quantified. ( d , e ) CD39, Atg5 and as a control β-actin protein expression in isolated KRas;Atg5 fl/+ and KRas;Atg5 fl/fl pneumocytes treated with the ( d ) HIF1α inhibitor 3-(2-(4-adamantan-1-yl-phenoxy)-acetylamino)-4-hydroxybenzoic acid methyl ester or left untreated and ( e ) the Nrf2 inhibitor Brusatol (100 nM) or the ROS scavenger N -acetyl- L -cysteine (5 mM). Protein lysates were analysed on day 4 by western blot. Quantifications of the CD39/β-actin ratios are shown for each lane. The inhibitors were present during the entire 4day culture period. Full size image Systemic treatment with the CD39 inhibitor polyoxometalate-1 (POM1) [46] reduces the oncogenesis-accelerating effect of autophagy deficiency without affecting the incidence of tumour initiation in autophagy-competent lung tumours ( Fig. 10a,b ). Since CD39 expression leads to the generation of adenosine [45] , we assessed whether blockage of adenosine receptors might also reduce the increased tumour incidence of KRas;Atg5 fl/fl mice. Treatment with the adenosine receptor antagonist PSB1115 (ref. 47 ) reduces the increased numbers of tumour foci in KRas;Atg5 fl/fl mice but not in the control KRas;Atg5 fl/+ littermates at 2 weeks after AdCre inhalation ( Fig. 10c,d ). Moreover, the CD39 inhibitor POM1 and the adenosinergic receptor agonist PSB1115 both abolished the increase in Treg infiltration of Atg5 -deficient tumours ( Fig. 10e,f ), supporting the notion that CD39 and adenosine act upstream of Treg to subvert immunosurveillance and to accelerate oncogenesis. These data support a connection between autophagy-repressed adenosinergic signalling, Treg accumulation, and tumour initiation. 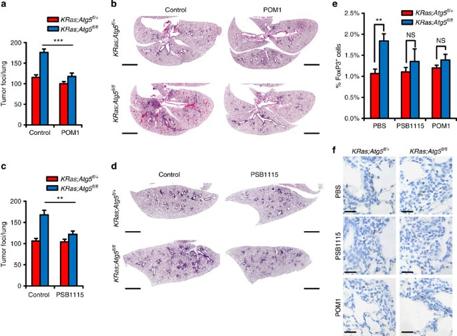Figure 10: Treatment of mice with CD39 and adenosine receptor blockers. (a) Quantification of numbers of hyperplastic lesions/per lung (mean values±s.e.m.) and (b) representative histological lung sections (haematoxylin and eosin (H&E) staining) ofKRas;Atg5fl/+andKRas;Atg5fl/flmice 2 weeks after AdCre inhalation treatedin vivoeither with either vehicle control or POM1 (intraperitoneally; i.p. 10 mg kg−1daily) to inhibit CD39 activity.n=4 per group. ***P<0.001 (χ2-test assessing the genotype effect in a generalized linear model with log link). Scale bars, 2 mm. (c) Quantification of numbers of hyperplastic lesions/per lung (mean values±s.e.m.) and (d) representative histological lung sections (H&E staining) ofKRas;Atg5fl/+andKRas;Atg5fl/flmice 2 weeks after AdCre inhalation treated either with either vehicle control or the adenosine receptor blocker PSB1115 (i.p. 10 mg kg−1daily).n=4 per group. **P<0.01 (χ2-test assessing the genotype effect in a generalized linear model with log link). Scale bars, 2 mm. (e,f) Representative immunohistochemistry and quantitative assessment of FoxP3+Tregs in lung tumours fromKRas;Atg5fl/+andKRas;Atg5fl/fllittermates treated with vehicle control or the CD39 blocker polyoxometalate-1 (POM1) and treated with vehicle or the adenosine receptor inhibitor PSB1115 (4-(2,3,6,7-tetrahydro-2,6-dioxo-1-propyl-1H-purin-8-yl)-benzenesulphonic acid potassium salt). Mice were killed 2 weeks after AdCre inhalation and their lungs were processed for immunohistopathology. Data are shown as mean percentages (±s.e.m.) of FoxP3+cells among total cell numbers in the tumour areas. Only cells within tumours were scored. At least four mice per genotype were analysed. Scale bars, 50 μm. **P<0.01. NS, not significant; (χ2-test assessing the genotype effect in a generalized linear model with logit link). Figure 10: Treatment of mice with CD39 and adenosine receptor blockers. ( a ) Quantification of numbers of hyperplastic lesions/per lung (mean values±s.e.m.) and ( b ) representative histological lung sections (haematoxylin and eosin (H&E) staining) of KRas;Atg5 fl/+ and KRas;Atg5 fl/fl mice 2 weeks after AdCre inhalation treated in vivo either with either vehicle control or POM1 (intraperitoneally; i.p. 10 mg kg −1 daily) to inhibit CD39 activity. n =4 per group. *** P <0.001 ( χ 2 -test assessing the genotype effect in a generalized linear model with log link). Scale bars, 2 mm. ( c ) Quantification of numbers of hyperplastic lesions/per lung (mean values±s.e.m.) and ( d ) representative histological lung sections (H&E staining) of KRas;Atg5 fl/+ and KRas;Atg5 fl/fl mice 2 weeks after AdCre inhalation treated either with either vehicle control or the adenosine receptor blocker PSB1115 (i.p. 10 mg kg −1 daily). n =4 per group. ** P <0.01 ( χ 2 -test assessing the genotype effect in a generalized linear model with log link). Scale bars, 2 mm. ( e , f ) Representative immunohistochemistry and quantitative assessment of FoxP3 + Tregs in lung tumours from KRas;Atg5 fl/+ and KRas;Atg5 fl/fl littermates treated with vehicle control or the CD39 blocker polyoxometalate-1 (POM1) and treated with vehicle or the adenosine receptor inhibitor PSB1115 (4-(2,3,6,7-tetrahydro-2,6-dioxo-1-propyl-1H-purin-8-yl)-benzenesulphonic acid potassium salt). Mice were killed 2 weeks after AdCre inhalation and their lungs were processed for immunohistopathology. Data are shown as mean percentages (±s.e.m.) of FoxP3 + cells among total cell numbers in the tumour areas. Only cells within tumours were scored. At least four mice per genotype were analysed. Scale bars, 50 μm. ** P <0.01. NS, not significant; ( χ 2 -test assessing the genotype effect in a generalized linear model with logit link). Full size image In various cancer models, autophagy has been reported either to inhibit or to accelerate oncogenesis and tumour progression [10] , [18] , [48] , making it paramount to accurately assess the role of autophagy in genetic models of tumour transformation. Our results indicate that Atg5 -dependent autophagy plays a dual role in lung cancer. Disabled autophagy initially increases the number of tumour foci and accelerates the transition from hyperplasia to adenomas. However, autophagy is then required for the efficient progression from adenoma to adenocarcinoma, indicating that disabled autophagy ultimately results in a reduction of tumour mass and improved survival of tumour-bearing mice. Autophagy has multiple effects on intracellular homoeostasis as well as on the relationship between cells and their microenvironment [49] . We found that disabled autophagy favours adenosinergic signalling via a Hif1α pathway, as well as the infiltration of tumours by Tregs, thus influencing inflammatory and immunosurveillance mechanisms that can stimulate and control carcinogenesis, respectively. Depletion of Tregs and inhibition of adenosinergic signalling both delayed the initiation of autophagy-deficient cancers. However, tumour cell autonomous effects of adenosinergic signalling cannot be excluded and should be explored in future in vivo experiments. Thus, autophagy functions to restrain the early steps of oncogenesis and the progression from hyperplasia to adenoma by effects on the tumour microenvironment. Disabled autophagy reportedly increases genomic instability [16] , but also enhances the DNA damage response (which is generally viewed as a brake of tumour progression) [34] , as it leads to the accumulation of dysfunctional mitochondria, reduced proliferation and an enhanced susceptibility to apoptotic or necrotic cell death. Our data reveal that, both in established tumours and in temporally controlled deletion experiments performed on primary pneumocytes, impaired autophagy results in a marked impairment of mitochondrial respiration, increased oxidative stress and an enhanced DNA damage response. Genetic inactivation of the tumour suppressor p53, which integrates multiple changes in bioenergetic metabolism [35] , reverted the impaired progression of autophagy-deficient adenomas to carcinomas. Of note, it has been recently reported that p53 also controls lung tumour progression in Atg7 -mutant mice [50] , corroborating our results. However, although the same lung tumour model was used, the phenotypes are different: the paper by Guo et al . [50] does not report accelerated oncogenesis for Atg7 -deficient tumours. Moreover, Guo et al . [50] did not observe any survival advantage of mice with Atg7 -null tumo u rs because of a diffuse lung inflammation causing their premature death. We failed to observe such an inflammatory phenotype in mice bearing Atg5 -null tumours. However, Guo et al . [50] observed that the absence of Atg7 delayed tumour progression and that this effect could be in part reverted by deletion of p53. Since the phenotype of Atg5 −/− tumours described here is different from that of Atg7 −/− cancers reported by Guo et al . [50] , putative autophagy-independent functions of either Atg5 or Atg7 should be explored in future experiments. In essence, autophagy plays a dual role in cancer, first as an inhibitor of initial oncogenesis and then as a facilitator of tumour progression. This complex dichotomy may have far-reaching implications for the avoidance and treatment of cancers that would, respectively, benefit from the induction and inhibition of autophagy. Generation of LSL-K-ras G12D ;Atg5 fl/fl mice Atg5 fl/fl mice were kindly given by Dr Noboru Mizushima. Exon 2 and 3 of Atg5 gene were targeted [24] . These mice were backcrossed for at least 10 generations onto a Balb/c background and then crossed to LSL-K-ras G12D mice [23] to generate LSL-K-ras G12D ;Atg5 fl/fl , LSL-K-ras G12D ;Atg5 fl/+ and LSL-K-ras G12D ;Atg5 +/+ mice. p53 fl/fl mice have been previously described [51] . Mouse genotypes were determined by PCR and, if required for confirmation, by DNA blot analysis. In all experiments, only littermate mice were used as controls. All mice were maintained according to the ethical animal licence protocol complying with the Austrian and European legislation. All experiments were approved by Bundesministerium for Wissenschaft und Forschung, Austria (BMWF-66.015/0013-II/3b/2012). Induction of lung cancer Inhalation of 6–8-week-old mice with AdCre viruses was performed as previously reported [29] . In brief, experimental animals were anaesthetized with 10% Ketasol/Xylasol and placed on a heated pad. An AdCre-CaCl 2 precipitate was produced by mixing 60 μl MEM, 2.5 μl AdCre (10 10 p.f.u. ml −1 ; University of Iowa, Gene Transfer Vector Core Iowa, USA) and 0.6 μl CaCl 2 (1 M) for each mouse and incubated for 20 min at room temperature (21–22 °C). Histology and immunohistochemistry Histological analysis of lung tumours was performed as previously described [29] . Briefly, 2 μm sections from at least three different planes of the lung were cut and stained with haematoxylin and eosin. Sections were scanned using a Mirax slide scanner and lung/tumour areas were automatically scored by an algorithm programmed and executed using the Definiens software suite and visually controlled in a blinded way. Immunhistochemical staining was done using an automatic staining machine (Leica Bond3) or manually processed. Sections were dehydrated and antigenic epitopes were retrieved using a 10-mM citrate buffer and microwaving for 10 min. Specimen were then incubated with rabbit polyclonal anti-γH2AX (Novus, NBP100-79967, 1:200 dilution), anti-Foxp3 (eBioscience, 13-5773, 1:100), anti-CD3ε (Santa Cruz, 101442, 1:100), anti-Ki67 (Novocastra, 1:200), anti-p62/SQSTM1 (Novus, NBP1-48320, 1:200), anti-Atg5 (Thermo Scientific, MA1378671, 1:100), anti-LC3I (Novus, NBP1-19167, 1:150), anti-Von Willebrand factor (DAKO, A0082, 1:100), anti-phospho-Chk2 (Novus, NB100-92502, 1:100), the macrophage marker anti-F4/80 (Santa Cruz, 59171, 1:150), anti-cleaved caspase-3 (Cell Signaling, 9661, 1:200), anti-HP1γ (Abcam, 66617, 1:100), and anti-PML (a kind gift of G. Ferbeyre, 1:100). Primary Ab staining was detected by peroxidase-conjugated anti-rabbit IgG (DAKO, P0448, 1:500). Terminal deoxynucleotidyl transferase dUTP nick-end labelling assays to detect DNA fragmentation was performed according to manufacturer’s instructions (Roche). Positive cells were counted on 20 randomly chosen tumour areas at × 400 magnifications in a double-blinded fashion. For PML quantification, images were captured with a Zeiss AxioImager Z1. Quantitative analysis was performed using HistoQuest software (TissueGnostics GmbH, Vienna, Austria; http://www.tissuegnostics.com ). Electron microscopy Freshly excised tissue was fixed in 2.5% glutaraldehyde in 0.1 mol l −1 sodium phosphate buffer, pH 7.4, for 1 h at room temperature. Subsequently, the samples were rinsed with the same buffer and post-fixed in 2% osmium tetroxide in the same buffer. After three washing steps with double-distilled H 2 O, the tissue was dehydrated in a graded series of ethanol and embedded in Agar 100 resin. Seventy nanometre sections (nominal thickness) were cut, post stained with uranyl acetate and lead citrate, and examined with an FEI Morgagni 268D (FEI, Eindhoven, The Netherlands) operated at 80 kV. Images were acquired using an 11 megapixel Morada charge-coupled device camera (Olympus-SIS). Mitochondrial bioenergetics Primary lung tumour pneumocytes were purified of 6 or 18 weeks after AdCre infection from 6 to 8-week-old male and female mice [29] . Following purification, 2 × 10 5 cells were seeded on XF24 cell culture plates coated with collagen type I. Seven to eight replicates per cell type were assayed in each experiment using Seahorse technology (Seahorse Bioscience). Cells were maintained in a 5% CO 2 incubator at 37 °C until the start of the experiment. On the day of the experiment, cells were washed and incubated in 675 μl XF Assay media (DMEM base 8.3 g l −1 , 3.7 g l −1 NaCl, phenol red, 25 mM glucose, 2 mM L -glutamine, pH 7.4) for 1 h at 37 °C. During the experiment, the oxygen concentration was measured every 6 min for a period of 2 min each. Oxygen consumption rate was calculated using the Fixed Delta technique for determining the slope. The first three cycles in the experiment were used to determine basal mitochondrial respiration rates. After recording basal respiration, successive injections of 0.4 μg ml −1 oligomycin, 0.4 μM FCCP (carbonyl cyanide- p -trifluoromethoxyphenylhydrazone) and 0.6 μM rotenone, each followed by three cycles determining Oxygen consumption rates, were carried out to determine the basal mitochondria respiration, ATP turnover, maximum mitochondrial respiratory capacity, non-mitochondrial respiration and proton leakage by calculating the region under the curve [52] . Western blotting and ELISA Western blotting was performed following standard protocols. The following primary Abs reactive to Atg5 (Cell Signaling, # 2630, 1:800 dilution), LC3I and LC3II (Cell Signaling, #2775, 1:1,000), p62/SQSTM1 (Cell Signaling, #8025, 1:1,000), cleaved caspase-3 (Cell Signaling, #9661, 1:1,000), cleaved caspase8 (Cell Signaling, #9748, 1:1,000), glyceraldehyde 3-phosphate dehydrogenase (Cell Signaling, #3638, 1:8,000), CD39 (Abcam, #128666, 1:600), Hif1α (Santa Cruz, sc-10790, 1:500) and β-actin (Sigma F3022, 1:10,000) were used. Membranes were incubated overnight with the primary Abs at 4 °C (diluted within 2.5% BSA in 1 × TBST buffer), washed three times in TBST for 15 min each and probed with horseradish peroxidase-conjugated secondary Abs (1:5,000, Promega) at room temperature for 1 h. Binding was detected by enhanced chemilumninescence (GE Healthcare, RPN2106). For detection of Cxcl5 in the sera, we used a Mouse Cxcl5 ELISA kit following the manufacturer’s instructions (Abcam, ab100719). For inhibitor experiments in primary pneumocytes, the Hif1α inhibitor 3-(2-(4-Adamantan-1-yl-phenoxy)-acetylamino)-4-hydroxybenzoic acid methyl ester (10 μM; Santa Cruz, sc-205346), the Nrf2 inhibitor brusatol [53] (100 nM; Chemical Book, #14907-98-3) and the ROS scavenger N -acetyl- L -cysteine (5 mM, Sigma, #A7250) were added to the cells 6 h after AdCre infection. Flow cytometry For FACS analysis, blood was removed from the lungs by injecting PBS in the right heart ventricle. Subsequently lungs were digested for 45 min at 37 °C in RPMI medium containing collagenase type 4 (600 U ml −1 ) and DNaseI (200 U ml −1 , both enzymes from Worthington). The following Abs were used for flow cytometry: anti-CD25 (PC61; BD Biosciences, 1:400 dilution), anti-CD4 (RM4-5, 1:800), anti-CD45 (30-F11, 1:500), anti-TCRβ (H57-597, 1:400), anti-TCRδ (GL3, 1:400), anti-CD11c (HL3, 1:400), anti-ICOS (C398.4A, 1:300), anti-LAG3 (C9B7W,1:300), anti-PD-1 (RMP1-30, 1:300; all Abs from Biolegend), anti-Foxp3 (FJK-16s, 1:400) and anti-LAP (TW7-16B4, 1:300; eBioscience). Single-cell suspensions were pre-incubated with anti-CD16/CD32 Fc receptor blocking Ab (clone 93; Biolegend, 1:200) and stained with the respective Abs. FoxP3 staining was performed according to the manufacturer’s instructions. FACS analysis was performed on a FACSCanto (BD Biosciences) and on an LSRFortessa (BD Biosciences) apparatus. Of note, we did not observe any difference in the lung infiltrates in Atg5 fl/fl and Atg5 fl/+ mice lacking the Cre-activatable KRas oncogene (and which do not develop tumours) after AdCre challenge, that is, the differences found in the immune infiltrates are clearly related to KRas-driven oncogenesis. Gene expression profiling Gene expression experiments were performed using Agilent SurePrint G3 Mouse GE 8 × 60K microarrays according to the manufacturers’ instructions. Two biological replicates and two technical replicates were performed for each sample. Reference samples comprised an equal mixture of the four experimental samples. For mRNAseq, total RNA was purified using RNAeasy mini Kit (Qiagen). Twice Poly-T selected RNA was isolated from 10 μg of total RNA and used as starting material for double-stranded complementary DNA synthesis. mRNAseq was performed at the CSF NGS Unit ( http://www.csf.ac.at/facilities/ngs/ ) using a Kapa library preparation kit. Final libraries were amplified using 15 PCR cycles, size selected by agarose gel for 200–600 basepair fragments and sequenced using 1 × 50 nucleotide reads on an Illumina HiSeq 2000. Differential expression analysis was performed using an empirical Bayes approach on linear models. Genes differentially expressed between KRas;Atg5fl /+ and KRas;Atg5fl /fl tumour cells were selected using a cutoff at a log2 fold-change>1 and a P -value of <0.05 (false discovery rate adjusted for multiple testing), and analysed for functional enrichment using IPA and GO. Complementary to the overrepresentation analysis of differentially expressed genes, we applied GSEA to identify GO gene sets (MSigDB v3.0 c5). The microarray and mRNAseq results are deposited under the ArrayExpress accession number E-MEXP-3653 and GEO accession number GSE48387 . microCT scanning Formaldehyde-perfused and fixed lungs were stained in a solution of 1% elemental iodine and 2% potassium iodide in distilled water for 3 days [54] . After staining, specimens were rinsed mounted in plastic tubes for microcomputed tomography (CT) scanning. Lungs were scanned using a SCANCO μCT 35 (SCANCO Medical AG, Brüttisellen, Switzerland) with a source energy of 70 keV and an intensity of 114 μA using a 0.2-mm copper filter. Projection images were recorded with an angular increment of 0.36°. Reconstructed microCT slices measured 1,024 × 1,024 pixels (voxel size=20 μm). Image stacks were imported into Amira 5.3 (Visualization Sciences Group, Mérignac Cedex, France) and filtered with a three-dimensional median filter (3 × 3 × 3 kernel). For segmentation of lung and tumour tissue, specific attenuation thresholds were used. For discriminating background from lung tissue an X-ray attenuation value of μ =0.3987 and for discriminating lung tissue from tumour tissue an attenuation value of μ =1.2776 was used. On the basis of segmentation, lung tissue and tumour volumes were calculated [54] . In vivo Treg depletion and inhibition of adenosinergic pathways Inactivation Tregs in vivo was performed as previously reported [42] , [43] . Briefly, anti-CD25 (500 mg per mouse, eBioscience, #16-0251), anti-FR4 (25 mg per mouse; Biolegend, #125102) or a rat IgG1 isotype control Ab (eBioscience, #16-4301; Biolegend, #400622) were injected once at day −1 before AdCre inhalation. 4-(2,3,6,7-Tetrahydro-2,6-dioxo-1-propyl- 1 H-purin-8-yl)-benzenesulphonic acid potassium salt (PSB1115, Tocris, #2009) and the ecto-nucleoside-triphosphate-diphosphohydrolase inhibitor POM1 (Tocris, #2689) were injected intraperitoneally at 10 mg kg −1 daily for the duration of the experiments. Quantitative reverse transcriptase–PCR Total RNA was prepared from tumours using the RNeasy Mini Kit (Qiagen) in accordance with the manufacturer’s instructions. Total RNA (2 μg) was subjected to reverse transcription using random hexamers (Roche) and SuperscriptII (Invitrogen) followed by quantitative PCR analysis. The following primers were used: Egr1: 5′-ATAGCAGCAGCAGCACCAG-3′ (forward) and 5′-GTCTCCACCATCGCCTTCTC-3′ (reverse); CXCL3: 5′-ACCAACCACCAGGCTACAG-3′ (forward) and 5′-CTTCTTGACCATCCTTGAGAGT-3′ (reverse); CXCL5: 5′-CGGTTCCATCTCGCCATTC-3′ (forward) and 5′-CGTTGCGGCTATGACTGAG-3′ (reverse); Gstm1: 5′-GCTCCTGGAATACACAGACTC-3′ (forward) and 5′-TCGATCAAGTAAGGCAGATTGG-3′ (reverse); Gstm3: 5′-CGCTTGCTCCTGGAATACAC-3′ (forward) and 5′-TGCTCTGGGTGACCTTGTG-3′ (reverse); and β-actin: 5′-GGCTGTATTCCCCTCCATCG-3′ (forward) and 5′-CCAGTTGGTAACAATGCCATGT-3′ (reverse). Statistics If not otherwise stated, all values are presented as means±s.e.m. For the Kaplan–Meier survival analysis, a log-rank test was performed. Tumour growth experiments were assessed by two-sided unpaired t -tests that are applied to proportions and to the corresponding log odds and a non-parametric two-sided and unpaired Wilcoxon test. Tumour growth was also modelled by applying Bayesian inference on a logistic growth model that also allowed us to assess Malthusian parameter (the maximum growth rates) and the limit proportions. Tumour progression was assessed by a cumulative link linear-mixed effects model to probe for significant dependency of overall progression on genotypes. Progression from hyperplasia to adenoma and from adenoma to adenocarcinoma was assayed by means of a generalized linear-mixed effects model with logit link. To improve robustness of our conclusions, we assessed genotype-related regression parameters for a significant deviation from zero and compared the model with the genotype regressor with an intercept-only model using a χ 2 -test. Quantifications of histological experiments were analysed by means of a generalized linear-mixed effects model with logit link by testing for non-zero regression coefficients and by using a χ 2 -test. Numbers of tumour foci were analysed by means of a mixed effects generalized linear model with log link by testing for non-zero regression coefficients and by using a χ 2 -test. Of note, we applied several tests to one data set to increase our confidence in the reported biological findings. P <0.05 was accepted as statistically significant. Accession codes : The microarray and mRNA sequencing results have been deposited in ArrayExpress and GEO databases under accession codes E-MEXP-3653 and GSE48387 , respectively. How to cite this article: Rao, S. et al . A dual role for autophagy in a murine model of lung cancer. Nat. Commun. 5:3056 doi: 10.1038/ncomms4056 (2014).